Caspase-2 is required for dendritic spine and behavioural alterations in J20 APP transgenic mice Caspases have critical roles in Alzheimer’s disease pathogenesis. Here we show that caspase-2 is required for the cognitive decline seen in human amyloid precursor protein transgenic mice (J20). The age-related changes in behaviour and dendritic spine density observed in these mice are absent when they lack caspase-2, in spite of similar levels of amyloid beta (Aβ) deposition and inflammation. A similar degree of protection is observed in cultured hippocampal neurons lacking caspase-2, which are immune to the synaptotoxic effects of Aβ. Our studies suggest that caspase-2 is a critical mediator in the activation of the RhoA/ROCK-II signalling pathway, leading to the collapse of dendritic spines. We propose that this is controlled by an inactive caspase-2/RhoA/ROCK-II complex localized in dendrites, which dissociates in the presence of Aβ, allowing for their activation and entry in the spine. These findings directly implicate caspase-2 as key driver of synaptic dysfunction in Alzheimer’s disease and offer novel therapeutic targets. Mice that carry transgenes encoding mutant human amyloid precursor protein (hAPP) develop many of the changes associated with Alzheimer’s disease (AD), including deficits in learning and memory, inhibition of long-term potentiation, loss of dendritic spines, profuse amyloid plaques and increased phosphorylation of the tau protein [1] . Changes similar to those seen in transgenic animals are replicated in vitro by treatment of cultured primary neurons with aggregated soluble amyloid beta (Aβ) oligomers, or in vivo by direct injection of Aβ oligomers into the hippocampus [2] , [3] . As neuronal death is usually not observed in hAPP transgenic mice, the non-apoptotic role of caspases (cysteine-aspartic proteases), in driving AD-related changes have remained largely unexplained. However, it is clear that caspases are crucial in contexts other than apoptosis, particularly in the maintenance of normal synaptic functions, whether in sculpting dendritic arborization and synapses [4] , [5] , guiding and pruning axons [6] , [7] , or in regulating long-term potentiation and long-term depression [8] , [9] . Disruption of normal synaptic function is one of the earliest events in AD [10] , [11] , raising the intriguing possibility that aberrant activation of caspases in AD brains may also have a pathogenic non-apoptotic role in driving these synaptic changes. Several caspases have been shown to be activated in human and in AD mouse model brains, including caspase-1, caspase-2, caspase-3, caspase-6 and caspase-9 (refs 12 , 13 , 14 , 15 , 16 ). Of all these caspases, however, our work has shown that only caspase-2 appears to be required for the apoptotic effects of Aβ in cultured hippocampal neurons. Hippocampal neurons for caspase-2 null mice are resistant to Aβ in spite of elevated levels of caspase-3, caspase-9 and the pro-apoptotic protein Smac/Diablo [17] , [18] . In the current study, we have revisited these earlier findings and investigated whether caspase-2 also has a significant role in mediating the effects of Aβ on synaptic plasticity and memory. We approached this question first in the J20 transgenic AD mouse model [19] . This mouse model features elevated levels of Aβ42, resulting from the introduction of the Swedish (K670N/M671L) and Indiana (V717F) hAPP mutations (that is, hAPPSwInd) and develop numerous plaques by the age of 5–7 months, as well as an age-dependent decline in learning in memory. We show that crossing the J20 mice with caspase-2 null mice results in the complete prevention of the memory impairments, as assessed by the radial-arm water maze (RAWM), and prevention of the loss of dendritic spine density typically observed in J20 mice, without significantly affecting amyloid load, inflammation and neuritic dystrophy. We further validated these results in an in vitro AD model using cultured primary hippocampal neurons where we show that downregulation of caspase-2 blocks the Aβ-mediated changes in dendritic spines. Additionally, our data suggest that caspase-2 may be a critical component in the activation and signalling of the Rho-GTPase RhoA, a critical regulator of dendritic spine morphology [20] , [21] . Taken together, these studies suggest that caspase-2 has a critical role in mediating the synaptic changes and memory alteration induced by Aβ in AD, and highlight caspase-2 as a potential target for AD therapy. Synaptotoxic effects of Aβ requires caspase-2 In order to determine if caspase-2 has a role in the subapoptotic effects of oligomeric Aβ at low (nM range) concentrations, in addition to its apoptotic role at higher (μM range) doses ( Supplementary Fig. S1a ), we exposed hippocampal neurons from wild-type (WT) rats to 300 nM Aβ with and without downregulation of caspase-2 and examined the effects on dendritic spine density and on levels of RhoA-GTP and ROCK-II. This resulted in a progressive decrease in spine density over the initial 24 h of exposure as well as increases in the levels of active RhoA-GTP and ROCK-II ( Fig. 1a,b and Supplementary Fig. S1b,c ). These effects were not seen in neurons exposed to the reverse Aβ peptide 42–1 ( Supplementary Fig. S2 ). When caspase-2 levels were decreased with an small interfering RNA (siRNA) by 65% ( Fig. 1f ), there was a partial blockade of the effect of Aβ on spine density and the levels of RhoA-GTP and ROCK-II, and complete protection against Aβ-induced spine reduction ( Fig. 1c–e , g ). Downregulation of caspase-3, caspase-8 and caspase-9 individually had no effect on spine density or on the levels of RhoA-GTP ( Fig. 2a,b,e–g ). As siRNA-mediated downregulation of each caspases was not complete ( Fig. 2f ), we wanted to rule out the possibility that residual caspase activity was responsible for the lack of protection. For that, we used commercially available irreversible caspase inhibitors to block caspase activity. Consistent with our siRNA results, only the caspase-2 inhibitor (VDVAD) blocked the effects of Aβ on dendritic spines, while the caspase-3 (DEVD) and caspase-8 (LEHD) inhibitors had no significant protective effect ( Fig. 2c,d ). These results were confirmed using hippocampal neurons from WT and caspase-2 null mice (Casp2KO). Before Aβ treatment, the spine density in neurons from each mouse line was similar. However, when the neurons were treated with Aβ, a significant loss of spines (~50% after 24 h) was seen in WT neurons but not in those derived from the Casp2KO mice ( Fig. 1h ). These experiments suggest that caspase-2 is not only critical for Aβ-induced apoptosis but also for the effects of Aβ on dendritic spines in cultured neurons. 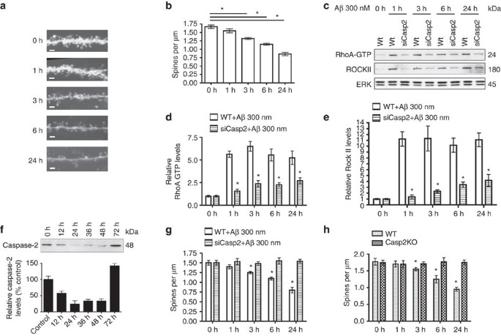Figure 1: Caspase-2 is required for Aβ-induced dendritic spine loss in hippocampal primary cultures. (a) Representative images of labelled dendrites over the course of 24 h after treatment with 300 nM Aβ. (b) Spine density (spines per μm) changes in rat primary hippocampal cultures treated with 300 nM Aβ for 24 h. Data presented as mean±s.e.m. (n=3 independent experiments, 150 dendrites per point, *P<0.05, one-way analysis of variance (ANOVA)). (c) Western blot analysis of primary hippocampal cultures pretreated for 12 h with 80 nM of Pen1-siRNA against caspase-2 showing no changes in RhoA-GTP or ROCK-II after a 24-h treatment with 300 nM Aβ. (d) Densitometric quantification of RhoA-GTP immunoblots. Data presented as the mean±s.e.m. (n=3 independent experiments, *P<0.05, two-tailed Student’st-test). (e) Densitometric quantification of ROCK-II immunoblots. Data presented as the mean±s.e.m. (n=3 independent experiments, *P<0.05, two-tailed Student’st-test). (f) Rat hippocampal primary cultures treated with 80 nM Pen1-siRNA against caspase-2 showing a time-dependent decrease in caspase-2 levels. Representative immunoblot for caspase-2 levels. Densitometric analysis of caspase-2 levels showing a 60% reduction by 12 h and persisting over 48 h. (g) Rat hippocampal primary cultures pretreated for 24 h with 80 nM Pen1-siRNA against caspase-2 show no decrease in spine density after treatment with 300 nM Aβ. Data presented as the mean±s.e.m. (n=3 independent experiments, 150 dendrites per point, *P<0.05, one-way ANOVA). (h) Hippocampal primary cultures derived from caspase-2 KO mice show resistance to 300 nM Aβ-induced spine loss, while WT neurons are sensitive to treatment. Data presented of the mean±s.e.m. (n=3 independent experiments, 150 dendrites per point, *P<0.05, one-way ANOVA). Figure 1: Caspase-2 is required for Aβ-induced dendritic spine loss in hippocampal primary cultures. ( a ) Representative images of labelled dendrites over the course of 24 h after treatment with 300 nM Aβ. ( b ) Spine density (spines per μm) changes in rat primary hippocampal cultures treated with 300 nM Aβ for 24 h. Data presented as mean±s.e.m. ( n =3 independent experiments, 150 dendrites per point, * P <0.05, one-way analysis of variance (ANOVA)). ( c ) Western blot analysis of primary hippocampal cultures pretreated for 12 h with 80 nM of Pen1-siRNA against caspase-2 showing no changes in RhoA-GTP or ROCK-II after a 24-h treatment with 300 nM Aβ. ( d ) Densitometric quantification of RhoA-GTP immunoblots. Data presented as the mean±s.e.m. ( n =3 independent experiments, * P <0.05, two-tailed Student’s t -test). ( e ) Densitometric quantification of ROCK-II immunoblots. Data presented as the mean±s.e.m. ( n =3 independent experiments, * P <0.05, two-tailed Student’s t -test). ( f ) Rat hippocampal primary cultures treated with 80 nM Pen1-siRNA against caspase-2 showing a time-dependent decrease in caspase-2 levels. Representative immunoblot for caspase-2 levels. Densitometric analysis of caspase-2 levels showing a 60% reduction by 12 h and persisting over 48 h. ( g ) Rat hippocampal primary cultures pretreated for 24 h with 80 nM Pen1-siRNA against caspase-2 show no decrease in spine density after treatment with 300 nM Aβ. Data presented as the mean±s.e.m. ( n =3 independent experiments, 150 dendrites per point, * P <0.05, one-way ANOVA). ( h ) Hippocampal primary cultures derived from caspase-2 KO mice show resistance to 300 nM Aβ-induced spine loss, while WT neurons are sensitive to treatment. Data presented of the mean±s.e.m. ( n =3 independent experiments, 150 dendrites per point, * P <0.05, one-way ANOVA). 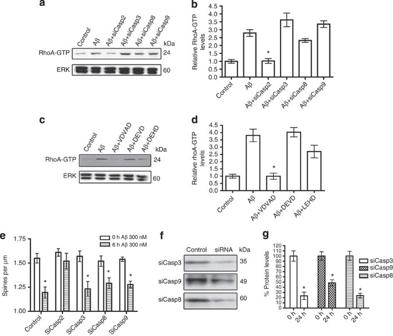Figure 2: Downregulation or inactivation of caspase-2 blocks Aβ-mediated effects on primary hippocampal cultures. (a) Representative western blot of hippocampal primary cultures treated for 1 h with 300 nM Aβ. The increase in RhoA-GTP levels is reversed by pretreatment with 80 nM Pen1-siRNA against caspase-2 but not with siRNA against caspase-3 (siCasp3), -8 (siCasp8) or -9 (siCasp9). (b) Densitometric analysis of RhoA-GTP levels from the immunoblots showing only the siCasp2 is able to block the changes observed from Aβ. Data presented as the mean±s.e.m. (n=3 independent experiments, *P<0.05, two-tailed Student’st-test). (c) Representative immunoblot from hippocampal primary cultures treated for 1 h with 300 nM Aβ; cultures were pretreated for 30 min with 0.5 μM of each caspase inhibitors: VDVAD (caspase-2); DEVD (caspase-3/7); LEHD (caspase-9). (d) Densitometric representation of RhoA-GTP levels of the immunoblot inc. Only caspase-2 inhibitor VDVAD blocks the Aβ-induced increase in RhoA-GTP. Data presented as the mean±s.e.m. (n=3 independent experiments, *P<0.05, two-tailed Student’st-test). (e) Spine density in primary hippocampal cultures pretreated for 24 h with siRNAs against caspase-2, -3, -8 and -9 and then treated for 6 h with 300 nM Aβ. Only siCasp2 protects against Aβ-mediated spine changes. Data presented as the mean±s.e.m. (n=3 independent experiments, 50 different dendrites per point; *P<0.05, one-way analysis of variance). (f) Representative immunoblots of primary cultures treated for 24 h with the respective siRNAs. (g) Densitometric analysis of caspase-3, -8 and -9 levels after 24 h treatment with the siRNA. Full size image Figure 2: Downregulation or inactivation of caspase-2 blocks Aβ-mediated effects on primary hippocampal cultures. ( a ) Representative western blot of hippocampal primary cultures treated for 1 h with 300 nM Aβ. The increase in RhoA-GTP levels is reversed by pretreatment with 80 nM Pen1-siRNA against caspase-2 but not with siRNA against caspase-3 (siCasp3), -8 (siCasp8) or -9 (siCasp9). ( b ) Densitometric analysis of RhoA-GTP levels from the immunoblots showing only the siCasp2 is able to block the changes observed from Aβ. Data presented as the mean±s.e.m. ( n =3 independent experiments, * P <0.05, two-tailed Student’s t -test). ( c ) Representative immunoblot from hippocampal primary cultures treated for 1 h with 300 nM Aβ; cultures were pretreated for 30 min with 0.5 μM of each caspase inhibitors: VDVAD (caspase-2); DEVD (caspase-3/7); LEHD (caspase-9). ( d ) Densitometric representation of RhoA-GTP levels of the immunoblot in c . Only caspase-2 inhibitor VDVAD blocks the Aβ-induced increase in RhoA-GTP. Data presented as the mean±s.e.m. ( n =3 independent experiments, * P <0.05, two-tailed Student’s t -test). ( e ) Spine density in primary hippocampal cultures pretreated for 24 h with siRNAs against caspase-2, -3, -8 and -9 and then treated for 6 h with 300 nM Aβ. Only siCasp2 protects against Aβ-mediated spine changes. Data presented as the mean±s.e.m. ( n =3 independent experiments, 50 different dendrites per point; * P <0.05, one-way analysis of variance). ( f ) Representative immunoblots of primary cultures treated for 24 h with the respective siRNAs. ( g ) Densitometric analysis of caspase-3, -8 and -9 levels after 24 h treatment with the siRNA. Full size image Memory impairments are absent in J20 mice lacking caspase-2 As experiments in cell culture are acute and cannot provide data on chronic effects or on the relationship of these changes to alterations in memory, we generated a new transgenic mouse line by crossing J20 mice [19] that overexpress mutant hAPP carrying the Swedish (K670N/M671L) and Indiana (V717F) hAPP mutations (that is, hAPPSwInd), with caspase-2 knock-out (Casp2KO) mice [22] , with both parental lines being on C57BL/6 backgrounds. Four distinct lines with four different genotypes were derived from these crosses: hAPP −/− /Casp2 +/+ referred to as WT; hAPP +/− /Casp2 +/+ referred to as J20; hAPP +/− /Casp2 −/− referred to as J20/Casp2KO and hAPP −/− /Casp2 −/− referred to as Casp2KO. We analysed these mice for dendritic spine morphology, amyloid accumulation, astrocytosis, microgliosis, dystrophic neurites and behaviour, as measured by RAWM. The animals were tested in the RAWM at 4, 9 and 14 months of age and then killed. The brains were examined by diOlistic labelling to determine dendritic spine density and the levels of active RhoA-GTP and ROCK-II were measured by western blotting. As differences in behaviour or in dendritic spine density could simply reflect differences in Aβ load or deposition, sections were also stained for plaques with an Aβ-specific antibody (6E10), and levels of soluble and acid-extractable Aβ were measured at each of the ages. As the results at 9 and 14 months were quite similar, we will focus our discussion on the changes at 14 months. At 4 months of age there were no detectable amyloid plaques in the brains of any of the 4 mouse lines and extractable Aβ levels showed no significant differences. No significant difference in task acquisition in RAWM was seen among the lines at 4 or 9 months of age ( Fig. 3a,b ). On the contrary, at 14 months of age the J20 animals and the Casp2KO animals were slower to learn the task than either WT or J20/Casp2KO animals ( Fig. 3c ). More importantly, only the J20 animals were impaired in task retention when compared with the three other lines at 4, 9 and 14 months of age ( Fig. 3d–f ). The differences in task retention were independent of motor, sensory or motivational changes among the different lines, as there were no observable changes in the latency to find a visible platform or in the swimming speed of these mice ( Fig. 3g,h ). 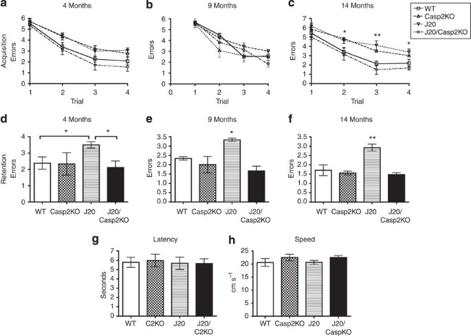Figure 3: J20/Casp2KO mice lack memory deficits seen in J20 mice. Mice from the four different lines were tested in the RAWM for spatial working memory at the ages of 4, 9 and 14 months. (a) At 4 months, there was no significant difference in task acquisition between WT, Casp2KO, J20 and J20/Casp2KO mice. (b) At 9 months, there was no significant difference in task acquisition between WT, Casp2KO, J20 and J20/Casp2KO. (c) At 14 months, J20 and Casp2KO mice showed impaired acquisition of the task as compared with WT and J20/Casp2KO littermates (7 male mice per group *P<0.05, two-way analysis of variance (ANOVA)). (d) During the retention trial, 4-month-old J20 mice showed a memory deficit compared with WT and J20/Casp2KO littermates, but not with Casp2KO (7 male mice per group, *P<0.05, two-way ANOVA). (e) At 9 months, J20 mice showed memory deficits compared with the other three lines: WT, Casp2KO and J20/Casp2KO (7 male mice per group, *P<0.05, two-way ANOVA). (f) Memory deficits persisted at 14 months of age (*P<0.05, **P<0.01, two-way ANOVA). (g,h) The four lines performed similarly in visible platform trials with regard to time to reach the platform (e) and speed (f). Figure 3: J20/Casp2KO mice lack memory deficits seen in J20 mice. Mice from the four different lines were tested in the RAWM for spatial working memory at the ages of 4, 9 and 14 months. ( a ) At 4 months, there was no significant difference in task acquisition between WT, Casp2KO, J20 and J20/Casp2KO mice. ( b ) At 9 months, there was no significant difference in task acquisition between WT, Casp2KO, J20 and J20/Casp2KO. ( c ) At 14 months, J20 and Casp2KO mice showed impaired acquisition of the task as compared with WT and J20/Casp2KO littermates (7 male mice per group * P <0.05, two-way analysis of variance (ANOVA)). ( d ) During the retention trial, 4-month-old J20 mice showed a memory deficit compared with WT and J20/Casp2KO littermates, but not with Casp2KO (7 male mice per group, * P <0.05, two-way ANOVA). ( e ) At 9 months, J20 mice showed memory deficits compared with the other three lines: WT, Casp2KO and J20/Casp2KO (7 male mice per group, * P <0.05, two-way ANOVA). ( f ) Memory deficits persisted at 14 months of age (* P <0.05, ** P <0.01, two-way ANOVA). ( g , h ) The four lines performed similarly in visible platform trials with regard to time to reach the platform ( e ) and speed ( f ). Full size image Synaptic changes are abrogated in J20 mice lacking caspase-2 Immediately after the behavioural analyses described above, the mice were killed to evaluate whether the differences in behaviour were reflected by changes in dendritic spine density and morphology. Spine density did not differ greatly at 4 months of age among genotypes ( Fig. 4a ). Moreover, there were no significant alterations in PSD95, Synapsin-1, RhoA-GTP or ROCK-II at 4 months of age ( Supplementary Fig. S3a,b ). However, analysis of spine morphology at this age revealed a significant decrease in the mushroom subtype in the J20 mice as compared with the WT and the J20/Casp2KO mice. The decrease in mushroom spines in the J20 animals is correlated with an increase in the stubby subtype that was not seen in the other lines ( Fig. 4c–e ). When similar studies were carried out at 14 months of age, dendritic spine density in the J20 animals was reduced to ~50% of the level seen in WT animals while the J20/Casp2KO animals, and the Casp2KO animals showed no loss of dendritic spines ( Fig. 4a,b ). To determine if these changes were limited to the hippocampus, we examined the frontal cortex where we found similar spine changes ( Supplementary Fig. S3c ). Similarly, biochemical analysis of the hippocampus at 14 months showed a reduction in both PSD95 and Synapsin-1 and an increase in RhoA-GTP and ROCK-II in the J20 animals ( Fig. 4f,g ). No changes in these markers were seen in the other three lines. 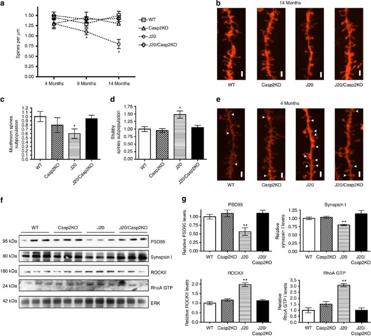Figure 4: Dendritic spine loss in J20 mice is reversed in J20/Casp2KO animals. Mice from each line (WT, Casp2KO, J20 and J20/Casp2KO) were analysed at 4, 9 and 14 months of age for spine changes. (a) J20 mice showed a significant decrease in spine density at 9 and 14 months of age compared with WT, Casp2KO and J20/Casp2KO mice. Data presented as the mean spine density ±s.e.m. (n=6 mice, 50 dendrites per mouse; *P<0.05, two-way analysis of variance (ANOVA)). (b) Images of DiI-labelled dendrites and spine morphologies in hippocampal neurons from 14-month-old mice of each line. (c) J20 mice showed a significant decrease in mushroom spine subpopulation at 4 months of age, while J20/Casp2KO mice showed same levels as WT. Histogram showing the relative number of mushroom-type spines compared with WT mice. Data presented as the mean density±s.e.m. (n=5 mice, 50 dendrites per mouse, *P<0.05, two-way ANOVA). (d) J20 mice showed a significant increase in stubby spine subpopulation at 4 months of age, while J20/Casp2KO mice showed similar levels as WT. Histogram showing the relative density of stubby-type spines compared with WT mice. Data presented as the mean density±s.e.m. (n=5 mice, 50 dendrites per mouse, *P<0.05, two-way ANOVA). (e) Images of DiI-labelled dendrites and spine morphologies in hippocampal neurons from 4-month-old mice of each line. (f) Representative western blots of hippocampal extracts from 14-month-old mice showing that alterations in synaptic and dendritic spine markers seen in J20 mice are absent in J20/Casp2KO mice (n=10 mice, **P<0.01, two-tailed Student’st-test). (g) Densitometric quantification of immunoblots inc. Levels of post- and pre-synaptic markers PSD95 and Synapsin-1 were reduced in J20 mice compared with WT and J20/Casp2KO mice (**P<0.01, two-tailed Student’st-test). Levels of ROCK-II and RhoA-GTP proteins were elevated in J20 mice compared with WT and J20/Casp2KO mice (**P<0.01, two-tailed Student’st-test). Histograms represent the densitometric mean±s.d. (n=10 mice). Figure 4: Dendritic spine loss in J20 mice is reversed in J20/Casp2KO animals. Mice from each line (WT, Casp2KO, J20 and J20/Casp2KO) were analysed at 4, 9 and 14 months of age for spine changes. ( a ) J20 mice showed a significant decrease in spine density at 9 and 14 months of age compared with WT, Casp2KO and J20/Casp2KO mice. Data presented as the mean spine density ±s.e.m. ( n =6 mice, 50 dendrites per mouse; * P <0.05, two-way analysis of variance (ANOVA)). ( b ) Images of DiI-labelled dendrites and spine morphologies in hippocampal neurons from 14-month-old mice of each line. ( c ) J20 mice showed a significant decrease in mushroom spine subpopulation at 4 months of age, while J20/Casp2KO mice showed same levels as WT. Histogram showing the relative number of mushroom-type spines compared with WT mice. Data presented as the mean density±s.e.m. ( n =5 mice, 50 dendrites per mouse, * P <0.05, two-way ANOVA). ( d ) J20 mice showed a significant increase in stubby spine subpopulation at 4 months of age, while J20/Casp2KO mice showed similar levels as WT. Histogram showing the relative density of stubby-type spines compared with WT mice. Data presented as the mean density±s.e.m. ( n =5 mice, 50 dendrites per mouse, * P <0.05, two-way ANOVA). ( e ) Images of DiI-labelled dendrites and spine morphologies in hippocampal neurons from 4-month-old mice of each line. ( f ) Representative western blots of hippocampal extracts from 14-month-old mice showing that alterations in synaptic and dendritic spine markers seen in J20 mice are absent in J20/Casp2KO mice ( n =10 mice, ** P <0.01, two-tailed Student’s t -test). ( g ) Densitometric quantification of immunoblots in c . Levels of post- and pre-synaptic markers PSD95 and Synapsin-1 were reduced in J20 mice compared with WT and J20/Casp2KO mice (** P <0.01, two-tailed Student’s t -test). Levels of ROCK-II and RhoA-GTP proteins were elevated in J20 mice compared with WT and J20/Casp2KO mice (** P <0.01, two-tailed Student’s t -test). Histograms represent the densitometric mean±s.d. ( n =10 mice). Full size image At 14 months of age, both the J20 and J20/Casp2KO animals showed approximately equal accumulation of amyloid plaques ( Fig. 5a,b ) and equal levels of expression of hAPP ( Fig. 5d ). No plaques were seen in the WT and Casp2KO animals and no hAPP expression was found. Levels of soluble and formic acid-extractable Aβ did not differ significantly between J20 and J20/Casp2KO mice ( Fig. 5e ). Although differences did not meet statistical significance, Aβ levels appeared be marginally lower in the J20/Casp2KO animals. GFAP staining revealed similar increases in astrocytosis both in the J20 and J20/Casp2KO as compared with the WT and Casp2KO animals ( Fig. 5a,c ). Increased tau phosphorylation is seen in the J20 animals but not in the J20/Casp2KO animals ( Supplementary Fig. S3d ). Staining for dystrophic neurites with SMI-312 (refs 23 , 24 ) and for microglia with Iba-1 (ref. 25 ) showed no significant difference between the J20 and J20/Casp2KO mice in the area surrounding the amyloid plaques ( Supplementary Fig. S4a–c ). 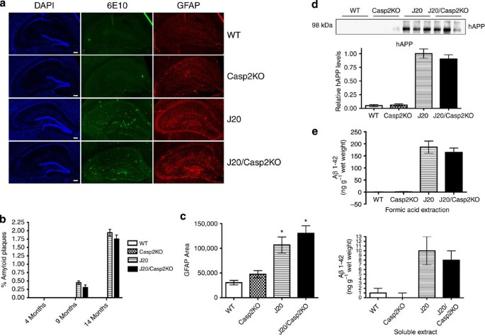Figure 5: APP levels, amyloid plaque load and astrogliosis in J20 and J20/Casp2KO mice are similar. At least six mice from each genotype were used to study APP levels and amyloid load. (a) Representative images at 14 months of hippocampal slices stained with DAPI, Aβ (6E10) and GFAP antibodies. (b) Amyloid plaque load in each of the four lines was quantified at 4, 9 and 14 months of age using ImageJ. Data presented as the percentage relative to the total area of the hippocampal slice. (c) GFAP immunopositive areas were quantified using ImageJ. Both J20 and J20/Casp2KO had elevated levels compared with WT or Casp2KO mice. Data are presented as the mean±s.d. (Five hippocampal slices per mouse were quantified, *P<0.05, one-way analysis of variance). (d) Representative western blot and densitometric analysis of protein extracts from mouse hippocampus showing similar levels of hAPP in both J20 and J20. Data presented as the mean±s.d. (e) Hippocampal Aβx–42levels in both insoluble and soluble fractions were measured by ELISA. There were no significant differences between J20 and Casp2KO mice. Data presented as the mean±s.d. (n=6 mice per line). Figure 5: APP levels, amyloid plaque load and astrogliosis in J20 and J20/Casp2KO mice are similar. At least six mice from each genotype were used to study APP levels and amyloid load. ( a ) Representative images at 14 months of hippocampal slices stained with DAPI, Aβ (6E10) and GFAP antibodies. ( b ) Amyloid plaque load in each of the four lines was quantified at 4, 9 and 14 months of age using ImageJ. Data presented as the percentage relative to the total area of the hippocampal slice. ( c ) GFAP immunopositive areas were quantified using ImageJ. Both J20 and J20/Casp2KO had elevated levels compared with WT or Casp2KO mice. Data are presented as the mean±s.d. (Five hippocampal slices per mouse were quantified, * P <0.05, one-way analysis of variance). ( d ) Representative western blot and densitometric analysis of protein extracts from mouse hippocampus showing similar levels of hAPP in both J20 and J20. Data presented as the mean±s.d. ( e ) Hippocampal Aβ x–42 levels in both insoluble and soluble fractions were measured by ELISA. There were no significant differences between J20 and Casp2KO mice. Data presented as the mean±s.d. ( n =6 mice per line). Full size image Caspase-2 and inactive RhoA form a complex It has been demonstrated that Aβ-treatment of neurons activates caspase-2 (ref. 26 ). The results presented above suggest that caspase-2 might have a role in the regulation of dendritic spine dynamics through RhoA. It has been reported that RhoB, a protein that is over 90% homologous with RhoA, is capable of binding to caspase-2 (ref. 27 ). To determine if a similar interaction underlies the role of caspase-2 in Aβ-mediated synaptic changes, we examined the interaction of these proteins in a series of co-immunoprecipitation studies from lysates of primary hippocampal neurons. We found that inactive RhoA (RhoA-GDP) but not active RhoA (RhoA-GTP) co-precipitated with caspase-2 ( Fig. 6a ). We were unable to directly immunoprecipitate RhoA-GDP or RhoA-GTP with the antibodies at our disposal and therefore turned to a cell-free system using recombinant caspase-2 and recombinant His-tagged inactive RhoA [His-RhoA] and His-tagged constitutively active RhoA [His-RhoA(Q63L)]. Consistent with our in vitro co-immunoprecipitation studies, only His-RhoA co-precipitated with caspase-2, but not constitutively active RhoA [His-RhoA(Q63L)]. Conversely, caspase-2 co-precipitated only with inactive His-RhoA, and not with active His-RhoA(Q63L) ( Fig. 6b,c ). Together, these results suggest a direct interaction between caspase-2 and inactive RhoA and not with active RhoA. This interaction does not appear to inhibit the activity of caspase-2, as the addition of inactive RhoA to recombinant active caspase-2 failed to block its activity as measured by fluorometric assay ( Supplementary Fig. S5a ). 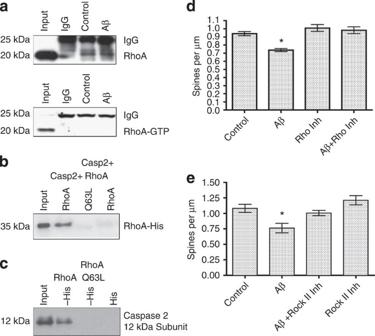Figure 6: Inactive RhoA and caspase-2 form a complex. (a) Immunoprecipitation of caspase-2 in rat hippocampal neuron extracts with showing co-precipitation of RhoA but not RhoA-GTP in both Aβ-treated and control cells. (b) RhoA-His but not RhoA(Q63L)-His co-precipitated with recombinant caspase-2 using anti-caspase-2 antibody. (c) Co-precipitation of the caspase-2 12 kDa subunit with RhoA-His but not with constitutively active RhoA(Q63L)-His using Dynabead His-Tag beads. (d) Synaptosomes from rat hippocampus were pretreated with bVAD-fmk before treatment with Aβ to trap active caspases. Treatment with either 300 nM or 1 μM Aβ led to activation of caspase-2. There was no caspase-2 activation in treated sonicated synaptosomes. (e) Inhibition of RhoA protects against Aβ-mediated spine loss. Rat hippocampal primary cultures were pretreated with 0.1 μg ml−1of Rho inhibitor or with PBS for 15 min before treatment with 300 nM Aβ for 5 h. Aβ treatment decreased spine number by 20% in cultures pretreated with PBS compared with control cultures while cultures pretreated with the Rho inhibitor, C3 transferase, showed no spine loss compared with controls. Data presented as the mean±s.e.m. (n=3 independent experiments, 150 dendrites per point, *P<0.05, one-way analysis of variance (ANOVA)). Figure 6: Inactive RhoA and caspase-2 form a complex. ( a ) Immunoprecipitation of caspase-2 in rat hippocampal neuron extracts with showing co-precipitation of RhoA but not RhoA-GTP in both Aβ-treated and control cells. ( b ) RhoA-His but not RhoA(Q63L)-His co-precipitated with recombinant caspase-2 using anti-caspase-2 antibody. ( c ) Co-precipitation of the caspase-2 12 kDa subunit with RhoA-His but not with constitutively active RhoA(Q63L)-His using Dynabead His-Tag beads. ( d ) Synaptosomes from rat hippocampus were pretreated with bVAD-fmk before treatment with Aβ to trap active caspases. Treatment with either 300 nM or 1 μM Aβ led to activation of caspase-2. There was no caspase-2 activation in treated sonicated synaptosomes. ( e ) Inhibition of RhoA protects against Aβ-mediated spine loss. Rat hippocampal primary cultures were pretreated with 0.1 μg ml −1 of Rho inhibitor or with PBS for 15 min before treatment with 300 nM Aβ for 5 h. Aβ treatment decreased spine number by 20% in cultures pretreated with PBS compared with control cultures while cultures pretreated with the Rho inhibitor, C3 transferase, showed no spine loss compared with controls. Data presented as the mean±s.e.m. ( n =3 independent experiments, 150 dendrites per point, * P <0.05, one-way analysis of variance (ANOVA)). Full size image Synaptotoxic effects of Aβ are RhoA/ROCK-II dependent Interestingly, we found that the activity of caspase-2 may be critical in mediating the effects of Aβ on cytoskeletal dynamics through its recently reported role in cleaving and activating the RhoA effector ROCK-II [28] . Indeed, exposure of primary hippocampal neurons to Aβ resulted in increased ROCK-II cleavage, generating a ~130 kDa fragment ( Supplementary Fig. S6a,b ), consistent with previous reports [28] , [29] . Depletion of caspase-2 in these neurons before Aβ treatment blocked ROCK-II cleavage, confirming the role of caspase-2 in cleaving ROCK-II. If RhoA and ROCK-II have critical roles in Aβ-mediated dendritic spine alterations, we would predict that inhibition of their activities should be able to block these changes. When primary hippocampal neuronal cultures were pretreated with the RhoA inhibitor, C3 transferase, or the ROCK-II inhibitor, Y27632, and then exposed to Aβ, the changes in spine density were abrogated ( Fig. 6d,e ). To determine if caspase-2 was involved more broadly in the control of RhoA-mediated signalling. We treated cells for 1 h with lysophosphatidic acid leading to the large increase in RhoA-GTP. Pretreatment of the cells with either siCasp2 or the commercially available caspase-2 inhibitor VDVAD partially blocks the increase in RhoA-GTP suggesting that caspase-2 is involved in regulating RhoA in response to diverse stimuli ( Supplementary Fig. S5b,c ). Caspase-2 regulates RhoA localization There is evidence that suggests that the distribution of RhoA may to be altered in AD and in AD mouse models [30] . We wondered whether Aβ could affect the localization of RhoA in neurons and whether caspase-2 has a role in this process. We exposed primary hippocampal neurons to Aβ and measured the localization of PSD95, RhoA and caspase-2 over the course of 24 h. ( Fig. 7a,b,f,g ). Before treatment with Aβ we found very low levels (~10%) of colocalization of RhoA with the synaptic marker PSD95 ( Fig. 7a,c ), suggesting that the majority of RhoA is found outside dendritic spines. After treatment with Aβ, there was a significant increase (~20%) after 6 h in the colocalization of RhoA and ROCK-II with PSD95, suggesting that Aβ treatment results in the recruitment of these proteins to dendritic spines, a translocation that has been suggested for RhoA in response to glutamate receptor modulation [31] . Although the ROCK-II increase at the spine is significant by 1 h and remains elevated over the treatment period, the RhoA translocation is more gradual. Similarly, before treatment, caspase-2 was mostly present in the dendritic shaft ( Fig. 7a,f ), but after treatment with Aβ, we observed a clear increase (~10%) in caspase-2 colocalization with PSD95 between 1 and 6 h post-treatment ( Fig. 7d ), suggesting that Aβ also triggers the translocation of caspase-2 to dendritic spines. When caspase-2 was downregulated in neurons before treatment with Aβ, the colocalization of RhoA and PSD95 was significantly diminished ( Fig. 7f,g ), consistent with a role for caspase-2 as a facilitator of RhoA translocation to dendritic spines after Aβ treatment. Aβ treatment also resulted in increased colocalization of caspase-2 with both RhoA and ROCK-II consistent with an interaction between caspase-2 and these proteins ( Fig. 7e,i ). Downregulation of caspase-2 before Aβ treatment significantly reduced the translocation of both RhoA and ROCK-II to the spines ( Fig. 8 ). 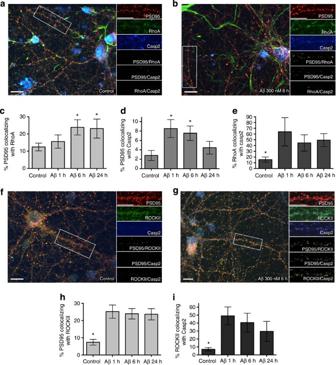Figure 7: RhoA, ROCK-II and caspase-2 translocate to spines following Aβ treatment. (a) Representative confocal images of vehicle-treated cultures stained for PSD95 (Red), RhoA (green) and caspase-2 (blue). Higher magnification examination of a dendritic segment revealed that both RhoA and caspase-2 were present mainly in dendritic shafts. Colocalization of proteins is represented in yellow (analysed with Volocity software; boxed areas showing enlarged dendritic segments. Scale bar, 10 μm). (b) Representative confocal images of culture hippocampal neurons treated for 6 h with Aβ 300 nM and stained for PSD95 (Red), RhoA (green) and caspase-2 (blue). (c) Quantification of colocalization of RhoA with PSD95, represented as the percentage of PSD95 puncta colocalized with RhoA. Data presented as the mean±s.e.m. (n=3 independent experiments, *P<0.05, one-way analysis of variance (ANOVA)). (d) Quantification of colocalization of caspase-2 with PSD95, represented as the percentage of the PSD95 puncta colocalized with RhoA. Data presented as the mean±s.e.m. (n=3 independent experiments, *P<0.05, one-way ANOVA). (e) Quantification of colocalization of caspase-2 with RhoA, represented as the percentage of the RhoA puncta colocalized with caspase-2. Data presented as the mean±s.e.m. (n=3 independent experiments, *P<0.05, one-way ANOVA). (f) Representative confocal image of an untreated hippocampal neuron stained for PSD95 (Red), ROCK-II (green) and caspase-2 (blue). Higher magnification of a dendritic segment revealed that both ROCK-II and caspase-2 were present mainly in dendritic shafts. Colocalization of proteins is represented in yellow (analysed with Volocity software; boxed areas showing enlarged dendritic segments. Scale bar, 10 μm). (g) Representative confocal image of a treated cultured hippocampal neuron (Aβ, 300 nM) stained for PSD95 (Red), ROCK-II (green) and caspase-2 (blue). (h) Quantification of colocalization of ROCK-II with PSD95, represented as the percentage of PSD95 puncta that colocalized with ROCK-II. Data presented as the mean±s.e.m. (n=3 independent experiments, *P<0.05, one-way ANOVA). (i) Quantification of colocalization of caspase-2 with ROCK-II, represented as the percentage of ROCK-II puncta colocalized with caspase-2. Data presented as the mean±s.e.m. (n=3 independent experiments, *P<0.05, one-way ANOVA). Figure 7: RhoA, ROCK-II and caspase-2 translocate to spines following Aβ treatment. ( a ) Representative confocal images of vehicle-treated cultures stained for PSD95 (Red), RhoA (green) and caspase-2 (blue). Higher magnification examination of a dendritic segment revealed that both RhoA and caspase-2 were present mainly in dendritic shafts. Colocalization of proteins is represented in yellow (analysed with Volocity software; boxed areas showing enlarged dendritic segments. Scale bar, 10 μm). ( b ) Representative confocal images of culture hippocampal neurons treated for 6 h with Aβ 300 nM and stained for PSD95 (Red), RhoA (green) and caspase-2 (blue). ( c ) Quantification of colocalization of RhoA with PSD95, represented as the percentage of PSD95 puncta colocalized with RhoA. Data presented as the mean±s.e.m. ( n =3 independent experiments, * P <0.05, one-way analysis of variance (ANOVA)). ( d ) Quantification of colocalization of caspase-2 with PSD95, represented as the percentage of the PSD95 puncta colocalized with RhoA. Data presented as the mean±s.e.m. ( n =3 independent experiments, * P <0.05, one-way ANOVA). ( e ) Quantification of colocalization of caspase-2 with RhoA, represented as the percentage of the RhoA puncta colocalized with caspase-2. Data presented as the mean±s.e.m. ( n =3 independent experiments, * P <0.05, one-way ANOVA). ( f ) Representative confocal image of an untreated hippocampal neuron stained for PSD95 (Red), ROCK-II (green) and caspase-2 (blue). Higher magnification of a dendritic segment revealed that both ROCK-II and caspase-2 were present mainly in dendritic shafts. Colocalization of proteins is represented in yellow (analysed with Volocity software; boxed areas showing enlarged dendritic segments. Scale bar, 10 μm). ( g ) Representative confocal image of a treated cultured hippocampal neuron (Aβ, 300 nM) stained for PSD95 (Red), ROCK-II (green) and caspase-2 (blue). ( h ) Quantification of colocalization of ROCK-II with PSD95, represented as the percentage of PSD95 puncta that colocalized with ROCK-II. Data presented as the mean±s.e.m. ( n =3 independent experiments, * P <0.05, one-way ANOVA). ( i ) Quantification of colocalization of caspase-2 with ROCK-II, represented as the percentage of ROCK-II puncta colocalized with caspase-2. Data presented as the mean±s.e.m. ( n =3 independent experiments, * P <0.05, one-way ANOVA). 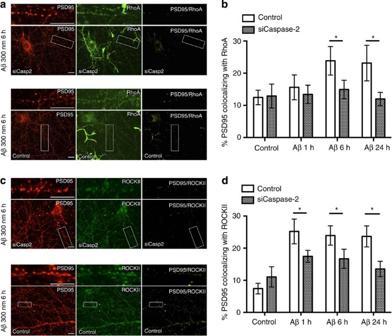Figure 8: Aβ-induced RhoA and ROCK-II translocation to dendritic spines is blocked by downregulation of caspase-2. (a) Representative confocal images of hippocampal cultures stained for PSD95 (Red) and RhoA (green), pretreated with siCasp2 or with vehicle (control) and treated for 6 h with 300 nM Aβ. Colocalization of proteins is represented in yellow (analysed with Volocity software; boxed areas showing enlarged dendritic segments. Scale bar, 10 μm). (b) Quantification of colocalization of RhoA with PSD95, represented as the percentage of PSD95 puncta colocalized with RhoA. Colocalization was measured before treatment with Aβ and at 1, 6 and 24 h after treatment. Data presented as the mean±s.e.m. (n=3 independent experiments, *P<0.05, one-way analysis of variance (ANOVA)). (c) Representative confocal image of a hippocampal neuron stained for PSD95 (Red) and ROCK-II (green) pretreated with siCasp2 or with vehicle and treated for 6 h with 300 nM Aβ. Colocalization of proteins is represented in yellow (analysed with Volocity software; boxed areas showing enlarged dendritic segments. Scale bar, 10 μm). (d) Quantification of colocalization of ROCK-II with PSD95, represented as the percentage of PSD95 puncta colocalized with ROCK-II. Colocalization was measured before treatment with Aβ and at 1, 6 and 24 h after treatment. Data presented as the mean±s.e.m. (n=3 independent experiments, *P<0.05, one-way ANOVA). Full size image Figure 8: Aβ-induced RhoA and ROCK-II translocation to dendritic spines is blocked by downregulation of caspase-2. ( a ) Representative confocal images of hippocampal cultures stained for PSD95 (Red) and RhoA (green), pretreated with siCasp2 or with vehicle (control) and treated for 6 h with 300 nM Aβ. Colocalization of proteins is represented in yellow (analysed with Volocity software; boxed areas showing enlarged dendritic segments. Scale bar, 10 μm). ( b ) Quantification of colocalization of RhoA with PSD95, represented as the percentage of PSD95 puncta colocalized with RhoA. Colocalization was measured before treatment with Aβ and at 1, 6 and 24 h after treatment. Data presented as the mean±s.e.m. ( n =3 independent experiments, * P <0.05, one-way analysis of variance (ANOVA)). ( c ) Representative confocal image of a hippocampal neuron stained for PSD95 (Red) and ROCK-II (green) pretreated with siCasp2 or with vehicle and treated for 6 h with 300 nM Aβ. Colocalization of proteins is represented in yellow (analysed with Volocity software; boxed areas showing enlarged dendritic segments. Scale bar, 10 μm). ( d ) Quantification of colocalization of ROCK-II with PSD95, represented as the percentage of PSD95 puncta colocalized with ROCK-II. Colocalization was measured before treatment with Aβ and at 1, 6 and 24 h after treatment. Data presented as the mean±s.e.m. ( n =3 independent experiments, * P <0.05, one-way ANOVA). Full size image Taken together, these results suggest that caspase-2 exerts at least a portion of its effects by controlling the localization, and perhaps the activity of the RhoA/ROCK-II signalling pathway leading to modulation of the actin cytoskeleton in the dendritic spines. Caspases have are most often thought of in connection with apoptosis. However, several lines of evidence have shown that caspases can also mediate a series of regulatory events in the mature nervous system designed to refine neuronal circuits, such as axon pruning and synapse elimination [4] , [5] , [6] , [7] . These processes are tightly regulated presumably by restricting the duration and location of caspase activation [32] . This implies that aberrant and mislocalized activation of caspases in living neurons could have detrimental effects on normal physiology and synaptic functions. Indeed, a number of caspases have been implicated in neurodegenerative diseases, including AD [12] , [13] , [14] , [15] , [16] . We previously demonstrated that caspase-2 was required, with caspase-3 being dispensable, for the apoptosis-inducing effects of Aβ in cultured hippocampal neurons [17] , [18] . Naturally, this led us to wonder whether caspase-2 was also involved in the synaptotoxic effects of Aβ. Using genetic, reverse genetic and pharmacological tools, both in primary neuronal culture and in the intact animal, we show that caspase-2 is the key regulator of dendritic spine density and morphology in response to Aβ. We found that knocking out caspase-2 in the J20 mice, completely prevented many of the age-dependent AD-like changes, including the memory deficits in performing the RAWM and the increase in phosphorylated tau protein (pTau). Knocking out caspase-2 in these mice completely abrogated the changes in spine morphology at an early age (4 months) and blocked the loss of dendritic spine density in older mice (14 months). It is interesting to note that the protective effects of knocking out caspase-2 in these animals occur without any significant changes in the levels of soluble Aβ or in the extent of plaque load. This raises an intriguing question as to whether AD-like changes in these animal models are due to Aβ or to overexpression of APP. The fact that these animals improve without much change to the Aβ burden suggests the possibility that much of the pathology is Aβ-independent. However, this oversimplifies the intimate relationship between Aβ and APP signalling. For example, while Aβ has been demonstrated to be highly toxic to cultured neurons [33] , APP itself appears to be necessary for this toxicity to occur [34] . The induction of APP signalling by its dimerization may in fact be sufficient to trigger neuronal death [35] . However, APP dimerization also leads to increased Aβ production [36] , [37] , [38] and to the formation of an APP-derived cytosolic toxic fragment, C31 (refs 39 , 40 , 41 ). Interestingly, blocking the formation of C31 also causes the reversal of cognitive impairments in J20 mice without affecting the levels of Aβ [42] , [43] . In our cell culture experiments, it is clear that Aβ causes changes similar to those seen in the mouse and the transduction of these signals requires APP cleavage [39] , [40] , [41] . In aggregate, these findings suggest a complex interrelation between accumulating Aβ and signalling by APP, its soluble APP ectodomains and its intracellular C-terminal fragments in mediating AD-like changes in animal models. Reducing the levels of any of these components eventually halts this complex signalling machinery allowing for the reversal of the associated cognitive decline [44] . The relative importance of elements of this pathway may differ with the stage of the disease and may explain the failure therapeutic strategies designed solely to decrease the levels of Aβ. The protective effects of knocking out caspase-2 were also recapitulated in a cellular model of AD-related synaptic dysfunction. Both siRNA and chemical inhibitor-mediated approaches to silence or inhibit caspase-2 proved successful in blocking the synaptotoxic effects of Aβ in cultured hippocampal neurons. Consistent with our previous report, silencing of caspase-3, caspase-8 and caspase-9 individually could not protect cultured neurons against Aβ exposure. Taken together, these results suggest that caspase-2 is a key factor in a novel mechanism regulating dendritic spine architecture and neural function that is ultimately mirrored in the behavioural tasks. These results are at variance with two recent reports implicating caspase-3 in the modulation of spine dynamics in similar mouse models [45] , [46] . It should be noted that the first of these studies relied on the detection of cleaved caspase-3 as a measure of activity. However, the cleavage of caspase-3 does not necessarily indicate that it is active in cells. Indeed, caspases are subject to regulation by a wide array of IAPs (inhibitor of apoptosis) and other regulatory proteins [18] , [47] . In the absence of specific intracellular reporters, in situ bVAD trapping of active caspases [48] remains the most reliable way to confirm that a given caspase is active. Furthermore, the exclusive reliance on pseudosubstrate inhibitors in that study precludes drawing any definitive conclusion as to the involvement of a specific caspase, as these inhibitors lack the required specificity [49] . The second report attempts to overcome several of these limitations by using the BIR domain of IAP proteins to specifically block caspase-3 activity. Although this domain does not affect caspase-2 activity, the analysis of the data is confounded by the fact that the BIR domain can also directly interact with cytoskeletal elements and block cytokinesis, as demonstrated in C. elegans [50] . Furthermore, the XIAP ring domain can also interact with Rho-regulatory protein, RhoGDI and promote the assembly of actin, a key component of dendritic spines [51] . Thus, it cannot be ruled out that the BIR-mediated protective effect is due to action on the actin cytoskeleton rather than on inhibition of caspase-3. The fact that depleting the protein levels of caspase-3 through RNAi in our studies fails to confer any protection against Aβ in neurons argues against a central role for caspase-3 in this process. The exact mechanism by which caspase-2 mediates the synaptotoxic effects of Aβ is an intriguing one and our results offer several important clues. Both caspase-2 and RhoA appear to reside outside of the spine head in the form of an inactive complex under normal conditions. This is supported by the fact that only inactive RhoA co-precipitates with caspase-2 and by the fact that we observe very little colocalization between them and the synaptic marker, PSD95. However, exposure to Aβ results in the activation of both caspase-2 and RhoA and the dissociation of the complex ( Fig. 6 ). In their active form, both RhoA and caspase-2 appear to enter the spine head, demonstrated by the fact that there is a significant increase in their co-localization with PSD95. One interesting observation is that downregulating caspase-2 is not sufficient for the translocation of RhoA to spines, suggesting that another anchor may be preventing this occurrence. A possible candidate for this role is the Rho–GDP dissociation inhibitor (RhoGDI), which sequesters Rho-GTPases from the membrane and prevents their interaction with guanine exchange factors. An interesting line for future investigations is to determine if both caspase-2 and Rho–GDI complex with RhoA-GDP at the same time or whether their binding is mutually exclusive. Once active RhoA and caspase-2 enter the spine head, they can affect the activity of one or more effectors to drive the collapse of the spines. One immediate candidate is the Rho effector ROCK-II, which has previously been shown to be activated by caspase-2-mediated cleavage [28] , and which we show to be cleaved in neurons treated with Aβ. In summary, our results clearly demonstrate that caspase-2 is an important mediator of Aβ synaptotoxicity in culture and in the intact animal. As caspase-2 expression is elevated in AD brain [52] , [53] , it is possible that inhibition of caspase-2, especially early in the course of AD, might prevent synaptic changes and memory deficits. The fact that we can protect neurons against Aβ with only a partial downregulation of caspase-2 suggests that therapeutic protection might be achieved without blocking critical actions of caspase-2 in other systems. Transgenic mice All animal studies were performed according to protocols examined and approved by the Animal Use and Care Committee of Columbia University. The J20 transgenic mouse line expresses a mutated human APP (hAPP: K670N/M671L and V717F) under the control of the platelet-derived growth factor promoter [19] , [54] . In our studies, we have used a J20 mouse line crossed to a C57BL/6 background (courtesy of Dr S-D Yan). Caspase-2 knockout (Casp2KO) mice [22] were also back-crossed to a C57BL/6 background. Double transgenic mice were obtained by crossing hemizygous transgenic mice J20 with Casp2KO mice. The first generation was crossed again with Casp2KO mice to generate the dual transgenic/null J20/Casp2KO mice. Transgenic mice were genotyped by PCR using oligonucleotides for human APP and caspase-2 with PuRe Taq PCR beads (Amersham). Male mice were divided into the following groups: WT, caspase-2 knockout (Casp2KO), J20 and J20/Casp2KO. Mice were tested blindly in the following experimental sequence: behaviour, biochemistry and histology. The complete sequence of behavioural tests was performed in the same mice at 4, 9 and 14 months of age. For each of the age groups, the complete sequence of behavioural tests required ~3 weeks and consisted of the RAWM test, and visible platform test. Immediately after behavioural testing at 14 month of age, mice were killed for DiOlistic labelling, biochemical and histological studies. Female mice were used only for the DiOlistic labelling, the biochemical, and histological studies and not for the behavioural studies. Radial-arm water maze The task has been described previously [55] . Each day of testing included four consecutive trials (A1–A4) and a fifth trial (R) 30 min after the fourth trial. The first four trials tested acquisition of the task, while the fifth trial tested retention memory (short-term memory). Each trial lasted 1 min. Errors were counted when the mouse went to an arm without platform or took more than 20 s to enter any arm of the maze. The number of errors in each trial in the last 3 days of testing was averaged and used for statistical analysis. DiOlistic labelling DiOlistic labelling was performed as previously described [56] . Briefly, mice were anaesthetized then fixed with 4% paraformaldehyde by transcardiac perfusion. Their brains were removed and sectioned coronally (300 μM) using a vibratome. Tissue sections were subsequently shot with DiI-coated particles using the Helios gene gun system. Hippocampal neurons were visualized using a spinning Disk Confocal Microscope and images were acquired with Perkin Elmer Volocity Software. Spines were counted manually in a double-blinded manner. NeuronStudio software was use to analyse the spine subtype populations. Histological studies Immunolabeling was done on 30 μm brain sections from the four genotypes. Staining was done using the anti Aβ antibody 6E10 (Covance), Aβ 1–42 (Abbiotech), Pan-Axonal Neurofilament SMI-312 (Covance), GFAP (Cell Signaling), anti microglia Iba-1 (Abcam). Plaque load and astrocytosis were quantified using ImageJ. Total plaque area was expressed as a percentage of the total hippocampal area. Astrocytosis was expressed as total area units. ELISA and western blot analysis Whole-frozen hippocampi were homogenized using a Teflon dounce homogenizer first in 150 mg ml −1 in 2% w/v sodium dodecyl sulphate (SDS) in water with protease inhibitors (Roche) to recover soluble amyloid. The sample was then centrifuged and the pellet homogenized in 70% formic acid in water to obtain the insoluble amyloid fraction. Homogenates were spun at 100,000 g for 1 h. Supernates were diluted in buffer EC (0.02 M sodium phosphate, pH 7.0, 0.2 mM EDTA, 0.4 M NaCl, 0.2% bovine serum albumin, 0.05% CHAPS) on ice. To obtain the soluble amyloid fraction and protein for western blotting, frozen hippocampi were homogenized using a Teflon dounce homogenizer in cell lysis buffer (Cell Signaling), sonicated briefly and centrifuged at 14,000 r.p.m. for 10 min. Aβ X–42 was measured by ELISA (Covance) following the manufacturers protocol. Immunoblotting was performed using the following polyclonal antibodies C-terminal APP (Calbiochem), caspase-2 (Abcam), PSD95 (Cell Signaling), Synapsin-1 (Chemicon) and ERK1 (Santa Cruz) and the monoclonal antibody for phospho-tau PHF13 (Cell Signaling). The caspase-2 polyclonal antibody was provided by the Troy laboratory [57] . Representative complete gels can be found in the Supplementary Information ( Supplementary Fig. S7 ). Immunofluorescence and microscopy Cells were fixed in paraformaldehyde (4%) in PBS for 10 min. Permeabilization was performed using 0.4% triton in PBS for 20 min. Cells were stained using the following antibodies PSD95 (Cell Signaling), Synapsin-1 (Chemicon) and caspase-2 (Millipore). Primary cultures were visualized using a spinning disk confocal microscope and images were acquired with Perkin Elmer Volocity software. Data analysis and statistics Immunoblotting, primary cultures of spine density, behavioural ELISA analysis and plaque burden analyses were performed with a two-tailed Student’s t- test. Mouse spine density data were analysed by two-way analysis of variance with age and genotype as independent variables. In all cases, P <0.05 was considered to be statistically significant. How to cite this article: Pozueta, J. et al. Caspase-2 is required for dendritic spine and behavioural alterations in J20 APP transgenic mice. Nat. Commun. 4:1939 doi: 10.1038/ncomms2927 (2013).